Structural rearrangements underlying ligand-gating in Kir channels Inward rectifier potassium (Kir) channels are physiologically regulated by a wide range of ligands that all act on a common gate, although structural details of gating are unclear. Here we show, using small molecule fluorescent probes attached to introduced cysteines, the molecular motions associated with gating of KirBac1.1 channels. The accessibility of the probes indicates a major barrier to fluorophore entry to the inner cavity. Changes in fluorescence resonance energy transfer between fluorophores, attached to KirBac1.1 tetramers, show that phosphatidylinositol-4,5-bisphosphate-induced closure involves tilting and rotational motions of secondary structural elements of the cytoplasmic domain that couple ligand binding to a narrowing of the cytoplasmic vestibule. The observed ligand-dependent conformational changes in KirBac1.1 provide a general model for ligand-induced Kir channel gating at the molecular level. Inward rectifier potassium (Kir) channels are encoded by members of a major structural K channel family. Each subunit contains a unique cytoplasmic 'Kir' domain, formed by the amino- and extensive carboxy- termini, through which these channels are physiologically regulated by a wide range of ligands [1] , [2] . For example, Kir1.x is gated by intracellular pH (refs 3 , 4 ), and Kir3.x (GIRKs) is opened by Gβγ subunits [5] , [6] , whereas Kir6.x (K ATP ) is closed by ATP [7] . All eukaryotic Kir channels share a common activatory ligand, phosphatidylinositol-4,5-bisphosphate (PIP 2 ), which again acts through binding to the Kir domain [8] , [9] , [10] . Despite the physiological significance of ligand-gating, the molecular motions associated with ligand-induced gating remain unclear. A class of prokaryotic Kir channel homologues, referred to as KirBac channels, have also been identified and characterized [11] , [12] , [13] , [14] , and crystal structures of full-length prokaryotic KirBac1.1 and eukaryotic Kir2.2 were first obtained in 2003 and 2009, respectively [15] , [16] . Kir channel crystal structures share high similarity to other K channel structures in the transmembrane regions, but are unique within the 'Kir' cytoplasmic domain [15] , [16] , [17] . Both eukaryotic Kir and KirBac channels therefore contain the appropriate 'Kir' domain for ligand-gating, although, in striking contrast to all eukaryotic Kir channels, KirBac1.1 is inhibited by PIP 2 (refs 13 , 18 , 19 ), potentially because of key structural differences in the linkers between the Kir domain and the transmembrane domains [8] , [19] , [20] . There is accumulating evidence that gating in many K channels, including inward rectifiers, requires a bending/rotating motion of the pore-forming transmembrane α-helices to remove the bundle crossing gate [21] , [22] , [23] , [24] , [25] , [26] . For KcsA, neutralization of negatively charged residues at acidic pH enhances the repulsion contributed by positively charged residues clustered at the bundle crossing, thereby stabilizing the channel in the open state [27] , [28] , [29] . Molecular dynamics simulations, mass spectrometric measurements, AFM techniques and GFP-based FRET approaches have also provided data consistent with the interpretation that ligand-dependent opening of Kir channels involves opening of the bundle crossing gate and rearrangement of the cytosolic domain [24] , [30] , [31] , [32] . Irrespective of where the ligand-operated gate is actually located, such studies have provided no information on the molecular motions of the Kir domain that underlie the gating, that is, the molecular motions that are induced by ligand binding. Recently, Clarke et al . [33] presented 11 KirBac3.1 crystal structures that demonstrate differences in ion occupancies within the selectivity filter, and differences within the cytosolic domain. We proposed a gating mechanism at the selectivity filter mediated by interaction between the cytoplasmic domain and the slide helix, although none of these structures actually demonstrate an opening of the bundle crossing that could support conduction, and it is not clear how the structural variants that are observed actually relate to gating states [34] . In the present work, we set out to examine gating motions within the KirBac1.1 channel protein that are definitively associated with ligand-gating, using PIP 2 as a ligand to drive channel closure. The data demonstrate specific motions of Kir domain β-sheets that result in narrowing of the cytoplasmic pore during PIP 2 -induced closure. A major pore barrier at the bundle crossing Wild-type KirBac1.1 contains no cysteines ( Supplementary Fig. S1 ) and thus provides a suitable model system for the introduction of cysteines that can be labelled with fluorescent tags. We first tested accessibility of substituted cysteines at different positions within the channel pore to Alexa Fluor 488 C5 maleimide (AF-488). The results ( Fig. 1a,c ) show that all substituted cysteines up to and including residue 150C are rapidly modified, indicating no barrier to the relatively bulky AF-488. There is only very slow modification of residues A147C and F149C, and no modification by AF-488 of cysteine residues that are actually within the inner cavity (A109C, T110C, I138C, T142C, G143C, V145C and F146C). In addition to a major restriction at the bundle crossing (immediately above residue 150), eukaryotic Kir crystal structures have revealed a secondary constriction at the so-called G-loop (that includes residue 264, Fig. 1e ), located just below the bundle crossing [35] , [36] , [37] . Our results indicate a major restriction at the bundle crossing, whereas the G-loop provides no detectable barrier to access of AF-488. 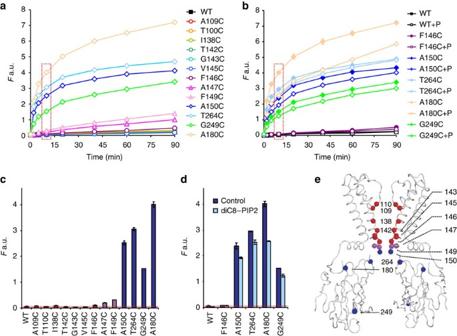Figure 1: Accessibility of KirBac1.1 channel pore lining residues. Time course (a, b) and 10 min time-point data (c, d, boxed ina, b) of Alexa-Fluor 488 C5 maleimide incorporation (F, a.u.) into cysteine-substituted KirBac1.1 mutants in the presence or absence of 10 μg ml−1diC8–PIP2 (mean±s.e.,n=3 in each case; error bars are smaller than symbol in most cases) (e) Ribbon diagram indicating accessibility of AF-488 to substituted cysteine residues. Alpha carbons of tested residues in this and subsequent figures are highlighted by spheres, with inaccessible residues coloured red, limited accessible (147 and 149) purple, and highly accessible blue. Figure 1: Accessibility of KirBac1.1 channel pore lining residues. Time course ( a, b ) and 10 min time-point data ( c, d , boxed in a, b ) of Alexa-Fluor 488 C5 maleimide incorporation ( F , a.u.) into cysteine-substituted KirBac1.1 mutants in the presence or absence of 10 μg ml −1 diC8–PIP2 (mean±s.e., n =3 in each case; error bars are smaller than symbol in most cases) ( e ) Ribbon diagram indicating accessibility of AF-488 to substituted cysteine residues. Alpha carbons of tested residues in this and subsequent figures are highlighted by spheres, with inaccessible residues coloured red, limited accessible (147 and 149) purple, and highly accessible blue. Full size image As discussed above, PIP 2 has an inhibitory effect on KirBac1.1 channel activity [13] , [19] , and modification rates of pore-lining cysteines within the cytoplasmic vestibule all dropped ~15% in the presence of 10 μg ml −1 diC8–PIP2 ( Fig. 1b,d ). The modification rate was even slower (~30%) at residue 180C that is located on the outer wall of the cytosolic domain. This residue is close to PIP 2 -binding sites recently identified in Kir2.2 and Kir3.2 by crystallography [8] , [35] , and, potentially, the reduced accessibility reflects shielding of 180C as a consequence of diC8–PIP2 binding. KirBac1.1 cysteine mutants are functional and PIP 2 sensitive Random labelling of mutant proteins with cysteine-reactive FRET donor/acceptor mixtures allows us to measure the gating-associated motions of labelled cysteines induced by PIP 2 . In the present work, cysteine residues were introduced at 21 different positions throughout the KirBac1.1 cytoplasmic domain ( Supplementary Fig. S1 ) and randomly labelled by EDANS C2 maleimide/DABCYL-plus C2 maleimide (E/D, R 0 =33 Å) or Alexa-Fluor-546 C5 maleimide/DABCYL-plus C2 maleimide (A/D, R 0 =29 Å). We previously showed that wild-type KirBac1.1 in phosphatidylethanolamine (POPE)/phosphatidylglycerol (POPG) (3:1) liposomes has high intrinsic open probability, but channel open probability is dramatically decreased by low levels of PIP 2 (refs 13 , 19 ). We examined the channel activity, and PIP 2 -sensitivity, of fluorophore-labelled KirBac1.1 cysteine mutants using a rubidium flux assay. Most fluorophore-labelled mutants are functional and remain sensitive to PIP 2 inhibition ( Fig. 2 ). Four mutants, including 177-AD, 186-AD, 228-AD and 306-ED were non-functional. Among these, 177-AD is apparently a consequence of the labelling, because 177-ED is still functional and PIP 2 sensitive. Residue 228 is located in the middle of the major β-sheet (βI, see below), whereas 186 is located at a subunit interface, and 306 is located at the extreme C-terminal end of the protein, in a small β-sheet region that is conserved among Kir channel members ( Supplementary Fig. S1 ). Structurally, these residues are all located far from the membrane interface and are unlikely to be involved in PIP 2 binding. Mutation and fluorophore-labelling may break their interactions with other residues, or block the ion conduction pathway, and the relevance of any PIP 2 -induced conformational changes at these sites to gating transitions, therefore, needs to be considered carefully (see Discussion ). We also noticed that 219C-AD is active but loses PIP 2 sensitivity. This residue is located in a connecting loop, and mutation or labelling may disrupt transduction of PIP 2 -triggered conformational changes, preventing closure of the channel pore ( Fig. 2 ). Consistent with this interpretation, this residue showed only minimal PIP 2 -dependent changes in FRET (see below). 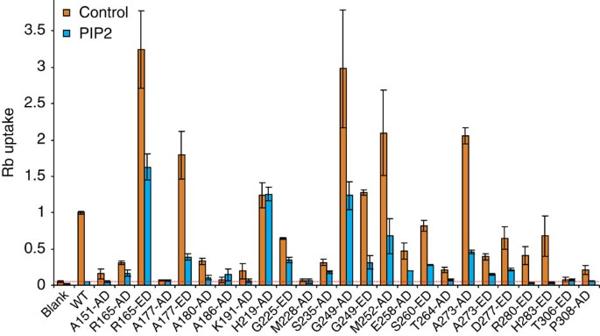Figure 2: Functional analysis of fluorophore-labelled KirBac1.1 cysteine-substituted mutants. Fluorophore-labelled KirBac1.1 mutants were reconstituted into liposomes (POPE:POPG=3:1) with or without 1.25% PIP2at protein/lipid ratio of 1:100 (w/w). The intraliposome buffer was 10 mM HEPES, 450 mM KCl and 4 mM NMDG, pH7.5, and the extraliposome buffer was 10 mM HEPES, 50 μM KCl, 400 mM sorbitol and 4 mM NMDG, pH7.5.86Rb+uptake was measured at 15 min and normalized against the maximal86Rb+uptake in the presence of valinomycin.86Rb+uptake of fluorophore-labelled mutants is shown as86Rb+flux relative to wild type (Rb uptake, mean±s.e.,n=3 in each case). Background level of86Rb+uptake (in liposomes with no protein) is marked by a red dashed line. Figure 2: Functional analysis of fluorophore-labelled KirBac1.1 cysteine-substituted mutants. Fluorophore-labelled KirBac1.1 mutants were reconstituted into liposomes (POPE:POPG=3:1) with or without 1.25% PIP 2 at protein/lipid ratio of 1:100 (w/w). The intraliposome buffer was 10 mM HEPES, 450 mM KCl and 4 mM NMDG, pH7.5, and the extraliposome buffer was 10 mM HEPES, 50 μM KCl, 400 mM sorbitol and 4 mM NMDG, pH7.5. 86 Rb + uptake was measured at 15 min and normalized against the maximal 86 Rb + uptake in the presence of valinomycin. 86 Rb + uptake of fluorophore-labelled mutants is shown as 86 Rb + flux relative to wild type (Rb uptake, mean±s.e., n =3 in each case). Background level of 86 Rb + uptake (in liposomes with no protein) is marked by a red dashed line. Full size image Movements of individual residues during PIP 2 -induced gating To investigate the gating-associated motions of the KirBac1.1 cytoplasmic domain, 21 cysteine mutants, labelled with E/D or A/D FRET pairs, were reconstituted into POPE/POPG (3:1) liposomes with or without 1.25% PIP 2 , and apparent FRET efficiencies were measured as described in the Methods. Unlabelled mutant protein, reconstituted into liposomes, was used as a control to subtract background fluorescence. Proteinase K was used to digest the protein and break the fluorescence resonance energy transfer pathway, thereby allowing measurement of maximum donor emissions ( Fig. 3a ) after 5–60 min. Four mutants were tested with both A/D and E/D pairs. In each case, the directional change of FRET was the same, although there were large differences in individual FRET efficiencies, which may be due to different R 0 of the FRET pairs, as well as the size and orientation of fluorophores ( Table 1 ). Predicted FRET efficiencies were calculated from absolute distances between residues in KirBac1.1 crystal structures (2WLL, 1P7B), assuming two- or four-fold symmetry (Methods and Supplementary Table S1 ). There was a significant correlation between FRET-reported inter-subunit distances and distances predicted by the KirBac1.1 crystal structure (2WLL) ( Fig. 3b ). Although the 2WLL crystal structure actually exhibits a slight two-fold symmetry, the correlation was essentially identical whether the measured FRET efficiencies were compared with the predicted efficiencies with either two-fold (ab) or four-fold symmetry (a = b ; Supplementary Fig. S2 ). 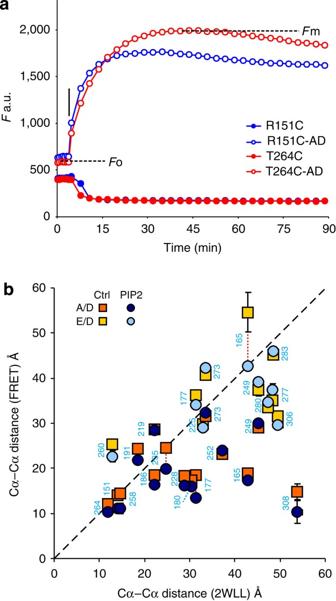Figure 3: FRET measurements reveal movements of individual residues during PIP2-induced closure. (a) Representative time course of FRET measurements by proteinase K-mediated donor dequenching. KirBac1.1 R151C and T264C tetramers were labelled by A/D mixtures, then reconstituted into liposomes (POPE:POPG=3:1). Proteinase K (0.08U per well) was added after 8 repeated readings (Fo) (T=5 min); Alexa-Fluor-546 emission (F, a.u.) was monitored until emission reached maximum (Fmax). (b) Cα–Cα distance between adjacent subunits of labelled residues predicted by FRET (mean±s.e.,n=6–9 in each case) versus those present in the KirBac1.1 (2WLL) crystal structure.RandPvalues of correlation are 0.51 (P<0.010), 0.54 (P<0.006) for Cα–Cα distances calculated from measured FRET efficiencies in the absence (control) and presence of 1.25% PIP2, respectively. Figure 3: FRET measurements reveal movements of individual residues during PIP 2 -induced closure. ( a ) Representative time course of FRET measurements by proteinase K-mediated donor dequenching. KirBac1.1 R151C and T264C tetramers were labelled by A/D mixtures, then reconstituted into liposomes (POPE:POPG=3:1). Proteinase K (0.08U per well) was added after 8 repeated readings ( F o ) ( T =5 min); Alexa-Fluor-546 emission ( F , a.u.) was monitored until emission reached maximum ( F max ). ( b ) Cα–Cα distance between adjacent subunits of labelled residues predicted by FRET (mean±s.e., n =6–9 in each case) versus those present in the KirBac1.1 (2WLL) crystal structure. R and P values of correlation are 0.51 ( P <0.010), 0.54 ( P <0.006) for Cα–Cα distances calculated from measured FRET efficiencies in the absence (control) and presence of 1.25% PIP 2 , respectively. Full size image Table 1 Changes of FRET efficiencies of labelled KirBac1.1 mutants in the presence or absence of PIP 2 . Full size table There is a good overall correlation between the FRET-reported distances and those predicted by the crystal structure ( Fig. 3b ). There is a systematic deviation in reported distances for E/D versus A/D pairs, that is, E/D reports wider distances (~20 Å), when both pairs are examined at the same residue. The side chains of these residues (165, 177, 249 and 273) all potentially orient towards the pore axis in the KirBac1.1 crystal structure. Because the spacer arm of EDANS is shorter than that of Alexa-Fluor 546 (by >10 Å), the A/D pair will report shorter distances than the E/D pair. There is significant deviation between FRET-reported distances and crystallographic predictions at two residues in particular, 165C-AD and 308C-AD. Residue 308 is located at the outside edge of the cytoplasmic domain, and we suggest that the lack of correlation may be a result of the flexible nature of this region or the relative orientation of fluorophores within the tetramer. The latter interpretation seems potentially correct for 165C; whereas the FRET-reported distance for 165C-AD is considerably less than that predicted from 2WLL, the 165C-ED-reported distance is actually well correlated ( Fig. 3b ) and, moreover, 165C-ED is functionally much more active than 165C-AD ( Fig. 2 ), suggesting a disruptive consequence of AD modification. Measured FRET efficiencies in the presence of PIP 2 show slightly better correlation with predicted FRET efficiencies from the KirBac1.1 crystal structure, consistent with the crystal structure being in a closed state. Residue motions suggest movements of secondary structures The KirBac1.1 cytoplasmic domain consists of two major β-sheets, one (which we refer to as βI, including residues 186, 191, 252, 258, 260, 264 and 273; Fig. 4a ) that is tilted ~45° relative to the membrane plane, and a second (βII, including residues 165, 177, 225 and 228; Fig. 4c ), that is approximately parallel with the pore axis. Small, but reproducible differences in FRET efficiencies (up to 15%), were detected for most residues in the presence and absence of PIP 2 ( Table 1 ). Comparison of FRET efficiencies in the presence (closed) and absence (open) of PIP 2 reveals important consistencies. First, in the presence of PIP 2 , all residues located at the top ends of βI move inwards relative to the central axis (264C, 260C, 258C, 186C and 191C), while residues at the bottom ends of βI (252C and 273C) and their attached short α-helix (249C and 277C) and β-sheets (280C and 283C) all move outwards. These data suggest a tilt motion of βI during PIP 2 -induced channel closure, with the top ends bending towards—and bottom ends bending away from—the pore axis ( Fig. 4a,b ). Second, all of the tested residues in βII and the associated loops and short helical stretches (219C, 225C, 228C, 235C, 180C, 177C, 165C, 306C and 308C) move inwards in the presence of PIP 2 , consistent with this whole region moving as a unit ( Fig. 4c,d ). Third, all cytoplasmic pore-lining residues (151, 264, 260, 258, 186, 191, 219 and 235), showed increased FRET efficiencies in the presence of PIP 2 , indicating that the cytoplasmic vestibule narrows throughout in the closed state ( Fig. 4 ), consistent with accessibility data ( Fig. 1 ). 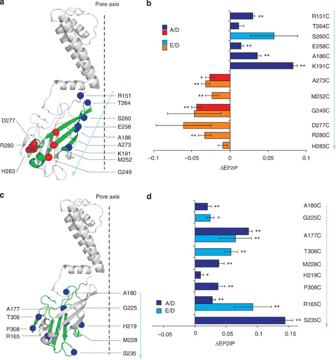Figure 4: Mapping FRET changes of individual residues to KirBac1.1 crystal structure suggest specific motions during gating. Changes of apparent FRET efficiencies of KirBac1.1 cysteine mutants in the large β-sheet (βI, panela, green andb) and small β-sheets (βII and associated loops, panelc, green andd) in presence versus absence of PIP2(ΔEPIP2, mean±s.e.,n=6–9 in each case). Inaandc, Cα of the labelled residue is highlighted by spheres; residues demonstrating inward motion in the presence of PIP2are coloured blue, those demonstrating outward motion are coloured red; the pore axis of KirBac1.1 is marked by dashed black line; amino acid residues in panelsbanddare listed from top to bottom, along the axis indicated by a solid blue line inaandc. Figure 4: Mapping FRET changes of individual residues to KirBac1.1 crystal structure suggest specific motions during gating. Changes of apparent FRET efficiencies of KirBac1.1 cysteine mutants in the large β-sheet (βI, panel a , green and b ) and small β-sheets (βII and associated loops, panel c , green and d ) in presence versus absence of PIP 2 (Δ E PIP2 , mean±s.e., n =6–9 in each case). In a and c , Cα of the labelled residue is highlighted by spheres; residues demonstrating inward motion in the presence of PIP 2 are coloured blue, those demonstrating outward motion are coloured red; the pore axis of KirBac1.1 is marked by dashed black line; amino acid residues in panels b and d are listed from top to bottom, along the axis indicated by a solid blue line in a and c . Full size image The growing number of K channels for which crystal structures are available (including KcsA [17] , MthK [21] , KvAP [38] , KirBac1.1 (ref. 15 ), Kv1.2 (ref. 39 ), NaK [40] , [41] and Kir2.2 (ref. 16 )) indicate that transmembrane domain structures are highly conserved. Crystallization of MthK in an open state provided the first direct view of an open K channel [21] , and revealed that removal of the major hydrophobic gate at the bundle crossing occurred by bending of pore forming α-helices away from the pore axis [21] , [22] . Similar structural changes have since been observed with open state crystal structures of KcsA [42] , [43] and NaK [41] . For Kir and KirBac channels, there is also strong evidence for ligand-gating occurring at or near the bundle crossing [25] , [26] , [44] , [45] . Our accessibility data indicate a significant barrier to fluorophore accessibility at the bundle crossing (F146), with enhanced accessibility of A150C immediately beneath the bundle crossing, and no significant barrier below this level. Rubidium flux assays indicate that PIP 2 significantly inhibits almost all labelled mutant channels ( Fig. 2 ), and our FRET studies reveal movements of multiple residues in the cytoplasmic domain in the presence of PIP 2 . In Rb flux assays, the potency of PIP 2 inhibition of labelled mutants ranges from ~40–99% ( Fig. 2 ), and, in most cases, inhibition will be incomplete, such that FRET-reported movements between open- and closed-conformations will be underestimations. In addition, uncertainties of fluorophore orientation factors preclude exact determinations of distances, but the direction of motion at each residue revealed by FRET measurements will be relatively robust. The qualitative patterns of directional movement (relative to the central axis of the channel) that then emerge ( Fig. 4 ) are consistent with essentially rigid-body motions of the major secondary structural elements within the cytoplasmic Kir domain, similar to the proposal of Nishida et al . based on observation of two distinct conformations of the KirBac1.3-Kir3.1 chimera cytoplasmic domain [46] . To visualize potential motions of the Kir domain, we generated 'cartoon' models for the open KirBac1.1 channel by modifying backbone coordinates of the closed KirBac1.1 (1P7B, Matlab, Mathworks Inc) in an attempt to match the constraints provided by the FRET measurements. Opening of the pore at the M2 helix bundle crossing was achieved by rotation and bending of TM2 at residue G134 (a potential hinge residue in K channels in general [21] , [47] ) and then coupled rigid-body motion of the cytoplasmic domain was applied. The degree of bending of TM2, and rigid translation of the C-terminal domain were varied to minimize disagreement with the FRET data. 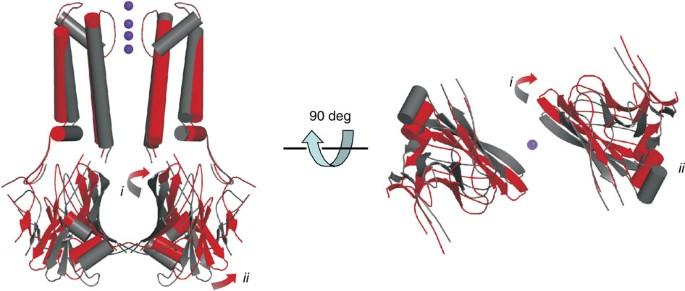Figure 5: 'Cartoon' model of ligand-gating of Kir channels. Views of closed (1P7B, grey) and 'open' (red) models of KirBac1.1 in (left) and from below (right) the plane of the membrane. Opening requires (i) outward twisting and tilting of βI, and (ii) outward motion of βII and associated short helices. For clarity, only two subunits are shown in each view. The unknown orientation factors of the fluorophores and potential perturbation effects of mutations and chemical labelling severely limit the resolution of the FRET measurements and prohibit unambiguous assessment of absolute distances, but the qualitative structural constraints obtained by FRET measurements are reasonably well met by the 'cartoon' open model shown in Figure 5 ( Supplementary Movie 1 ). The model was generated by tilting of βI, with the top end moving away from, and the bottom end towards, the pore axis ( i ), which widens the upper end of the cytoplasmic vestibule, and anticlockwise twist of βII leads to changes in the subunit interfaces and movement of βII away from the central axis ( ii ), which widens the cytoplasmic pore. The directional movements indicated by the FRET measurements are replicated for 19 out of 21 residues ( Table 1 ), and are consistent with results obtained from other biochemical and biophysical studies on Kir channel open state conformations [30] , [44] , [45] , as well as predictions of molecular dynamic simulation studies [24] , [47] , [48] , [49] . Figure 5: 'Cartoon' model of ligand-gating of Kir channels. Views of closed (1P7B, grey) and 'open' (red) models of KirBac1.1 in (left) and from below (right) the plane of the membrane. Opening requires ( i ) outward twisting and tilting of βI, and ( ii ) outward motion of βII and associated short helices. For clarity, only two subunits are shown in each view. Full size image Eukaryotic and prokaryotic Kir channels have distinct and opposite responses to PIP 2 : while KirBac1.1 is closed by PIP 2 binding, all eukaryotic Kir channels are opened by PIP 2 . The different response to PIP 2 is likely to depend on critical differences in binding site orientation or on coupling of binding to the Kir domain gating machinery. Different structures of the loops that link the transmembrane and cytoplasmic domains constituting the PIP 2 binding pocket are likely to be important [15] , [16] . Indeed, a recently solved crystal structure of PIP 2 -bound Kir2.2 indicates key interacting residues that are absent from the linker loop of KirBac1.1 (ref. 8 ). A second PIP 2 -bound Kir3.2 structure reveals binding at a similar location [35] , and, moreover, PIP 2 binding, which leads to channel activation in Kir3.2 channels, causes a twist in the major (β1) β-sheet that is qualitatively quite similar to that which we predict in the (PIP 2 -unbound) 'open' KirBac1.1. The eukaryotic Kir family exhibits sensitivity to a remarkably broad range of cytoplasmic ligands that are all likely to converge on similar conformational responses. Each subfamily from Kir1 to Kir7 has been shown to be activated by PIP 2 (refs 50 , 51 , 52 , 53 , 54 , 55 , 56 ), and biophysical analyses demonstrate that the unique ligands for different subfamilies (pH in Kir1 and Kir4; Na and G-protein βγ subunits in Kir3; ATP in Kir6) are convergent on the same process, such that kinetic models of gating implicitly involve the same gate as that activated by PIP 2 . This leads us to speculate that open-closed motions that we detect in the present study will be replicated in the ligand-induced gating of all eukaryotic inward rectifiers. DNA manipulation and protein expression DNA manipulation, expression and purification of KirBac1.1 cysteine substitution mutants are essentially as described previously [12] , [19] , [57] except for changing the gel filtration buffer to 20 mM HEPES with 150 KCl and 5 mM DM, pH 7.5. Tetramer fractions were collected and concentrated to 3 mg ml −1 for chemical labelling with the maleimide form of fluorophore pairs. Cysteine-substituted KirBac1.1 mutants were labelled with EDANS C2 maleimide/DABCYL-plus C2 maleimide (E/D, ANASPEC), at protein:E:D ratio of 1:10:10, or with Alexa-Fluor-546 C5 maleimide (Invitrogen)/DABCYL-plus C2 maleimide (A/D) at a protein:A:D ratio of 1:2.5:10. Labelling reactions were performed at room temperature for 1 h,and, then, proteins were loaded onto a 5 ml Hitrap desalting column (GE Healthcare) to remove free probe. Labelled protein samples were collected and concentrated to 1.0 mg ml −1 (KirBac1.1-A/D) or 3.0 mg ml −1 (KirBac1.1-E/D) for reconstitution. Accessibility assay using Alexa Fluor 488 C5 maleimide Accessibility assays were performed at room temperature using labelling buffer containing ~400–500 ng of KirBac1.1 in labelling buffer (20 mM Hepes, 150 mM KCl, 5 mM DM, pH7.5) were immobilized on His-Sorb plates (Qiagen), and, then, the assay was started by adding AF-488 at final protein:probe ratio of 1:50, in the presence or absence of 10 μg ml −1 of diC8–PIP 2 . Free probes were removed by washing with labelling buffer (3×) and incorporation of AF-488 was monitored by emission at 525 nm with excitation wavelength of 485 nm. KirBac1.1 wild-type protein was used as control to estimate and subtract nonspecific labelling. Reconstitution of labelled KirBac1.1 into liposomes Lipids (3:1 POPE:POPG, Avanti Polar Lipids) were solubilized in buffer A (150 mM KCl, 20 mM HEPES, pH 7.5) containing 37 mM CHAPS with or without 1.25% PIP 2 (w/w). The KirBac1.1 cysteine mutants form tetrameric proteins with one cysteine in each monomer. Combinatorially, labelling with E/D or A/D FRET pairs gives six different configurations of donor and acceptor labels, four of which will have at least one donor and acceptor within a given tetramer ( Supplementary Table S1 ). The lipids were mixed with fluorophore-labelled protein at a ratio of 100:3 for KirBac1.1-E/D and 100:1 for KirBac1.1-A/D. The lipid/protein mixture was incubated for 20 min at room temperature, and then loaded onto a Sephadex G-50 column pre-equilibrated with buffer A to remove CHAPS and to obtain reconstituted proteoliposomes. FRET Measurements FRET experiments were performed using a Synergy 2 fluorescence reader with excitation/emission wavelengths of 360/460 nm for KirBac1.1-E/D and 540/570 nm for KirBac1.1-A/D. Following 8 repeated readings, proteinase K solution was added to the proteoliposome sample at a final concentration of 0.08 U per well. Fluorescence was monitored until reaching a new stable plateau. Unlabelled protein samples were reconstituted into liposomes with or without PIP 2 as controls to measure background fluorescence intensities. Fluorescence emission was measured before ( F o ) and after proteinase digestion ( F max ). The apparent FRET efficiency ( E app ) is then given by the ratio of the quenched donor emission to the maximum donor emission: Rubidium flux assay Fluorophore-labelled KirBac1.1 cysteine mutants were reconstituted into liposomes containing 3:1 POPE:POPG with or without 1.25% PIP 2 , at protein:lipid ratio of 1:100, as described by Enkvetchakul et al . [12] , [19] The KCl concentration inside and outside of the liposome was 450 mM and 50 μM, respectively. Rubidium uptake over 15 min was measured and normalized to valinomycin-dependent maximum uptake. All data are presented as mean±s.e. from three independent repeats. Data analysis For fluorescence measurements, data are expressed as mean±s.e. of multiple independent labelling and reconstitution experiments. Error propagation was used to calculate s.e. in Fig. 4 . For calculating the apparent FRET efficiencies predicted by the crystal structure of KirBac1.1 (2WLL, or the 'open' structure model) in Table 1 and Supplementary Fig. S2 , the distances between α-carbon of FRET-measured residues at two adjacent subunits were used. For a tetramer with multiple donor and acceptor present, apparent FRET efficiencies ( E app ) were calculated based on resonance energy transfer rate theory as described in detail by Cheng et al . [58] ( Supplementary Table S1 ) using the following equation: with the assumption that both donor and acceptor fluorophores are randomly incorporated into the KirBac1.1 tetramer. The Cα distance, predicted by experimentally measured apparent FRET efficiencies in Figure 3b, was obtained using the same FRET model by setting a = b . ( Supplementary Table S1 ). How to cite this article: Wang, S. et al . Structural rearrangements underlying ligand-gating in Kir channels. Nat. Commun. 3:617 doi: 10.1038/ncomms1625 (2012)